Single rhodium atoms anchored in micropores for efficient transformation of methane under mild conditions Catalytic transformation of CH 4 under a mild condition is significant for efficient utilization of shale gas under the circumstance of switching raw materials of chemical industries to shale gas. Here, we report the transformation of CH 4 to acetic acid and methanol through coupling of CH 4 , CO and O 2 on single-site Rh 1 O 5 anchored in microporous aluminosilicates in solution at ≤150 °C. The activity of these singly dispersed precious metal sites for production of organic oxygenates can reach about 0.10 acetic acid molecules on a Rh 1 O 5 site per second at 150 °C with a selectivity of ~70% for production of acetic acid. It is higher than the activity of free Rh cations by >1000 times. Computational studies suggest that the first C–H bond of CH 4 is activated by Rh 1 O 5 anchored on the wall of micropores of ZSM-5; the formed CH 3 then couples with CO and OH, to produce acetic acid over a low activation barrier. CH 4 has been one of the inexpensive energy resources since the maturation of hydraulic fracturing technology. So far, most processes of transformation of CH 4 to intermediate compounds for chemical industries including steam or dry reforming, partial oxidation, and oxidative coupling are performed at high temperatures. One side effect of these processes is the deactivation of catalysts due to coke formation [1] , [2] . Another is the input of huge amount of energy since they are performed at high temperatures. Thus, activation of C–H of CH 4 at a low temperature is necessary in order to transform shale gas to intermediate compounds of chemical industries in an energy-efficient manner [3] , [4] , [5] , [6] , [7] , [8] , [9] . Acetic acid is one of the important intermediates of chemical industries. The global demand is 6.5 million metric tons per year (Mt/a). Currently, it is produced from methanol carbonylation, in which CO reacts with methanol to form acetic acid. However, methanol is synthesized from CO and H 2 , which are produced from steam reforming processes of either methane or coal at high temperatures [10] . Replacement of the current high-temperature catalysis toward production of acetic acid with catalysis at low temperatures would be feasible if a catalytic process on a heterogeneous catalyst could efficiently, directly transform CH 4 to acetic acid under a mild condition. Transformations of methane to methanol and acetic acid on isolated palladium and rhodium atoms anchored in zeolite in liquid solution were simultaneously explored in our group since early 2012. We reported oxidation of methane to form methanol on Pd 1 O 4 anchored in ZSM-5 in aqueous solution at low temperature in 2016 [11] . Other than the mild oxidation of CH 4 to CH 3 OH with supported isolated Pd atoms anchored in ZSM-5, we have simultaneously studied oxidization of methane through coupling with CO and O 2 to methanol and acetic acid on isolated Rh atom anchored in ZSM-5 since 2012 and the Rh 1 O 5 /ZSM-5 catalyst was synthesized and its high activity was confirmed and its structure was identified before summer of 2014. Formation of single sites is a significant approach to developing catalyst toward high catalytic activity and selectivity [11] , [12] , [13] , [14] , [15] , [16] , [17] . Separately anchoring catalytic sites (M 1 ) on an oxide support (M 1 /A x O y ) tunes the electronic state of catalytic sites of metal atoms (M 1 ), which are typically continuously packed on surface of a metal nanoparticle or periodically located in a surface lattice of a metal oxide nanoparticle (M x O y ). Compared to continuously packed M atoms on surface of a metal nanoparticle (····M-M-M····) and periodically packed M cations in surface lattice of a metal oxide nanoparticle (···O-M 1 -O-M 1 * -O-M 1 -O-M 1 -O ····), these isolated cation sites (M 1 * ) anchored on surface of a substrate oxide (A a O b ), ···O-A-O-M 1 * -O-A-O-A, exhibit a distinctly different coordination of M atoms. Thus, those isolated cations (M 1 ) could exhibit a catalytic performance distinctly different from a metal oxide nanoparticle (M x O y ) or a metal nanoparticle. We separately anchored Rh cations on the internal surface of micropores of an aluminosilicate, H-ZSM-5 through ion exchange between Rh 3+ in solution and H + on the internal surface of micropore, similar to the isolated palladium atoms in ZSM-5 [11] . As these Bronsted sites are typically isolated, Rh 3+ cations can be separately anchored on Bronsted sites. Production of acetic acid through coupling CH 4 with CO and O 2 (2CH 4 +2CO+O 2 →2CH 3 COOH) is efficiently catalyzed by these singly dispersed Rh sites, Rh 1 O 5 . Different from rhodium atoms anchored on nonporous silicate and other nonporous oxide, this heterogeneous catalyst exhibits high activity in transforming CH 4 to acetic acid, about 0.1 CH 3 COOH molecules per Rh site per second with a selectivity of ~70% for production of acetic acid. Isotope-labeled experiments using 13 CH 4 and 13 CO show that CH 3 of CH 3 COOH forms from activation of CH 4 to CH 3 and C=O of CH 3 COOH from insertion CO to Rh-OH. Density functional theory (DFT) calculation suggests that activation of C–H of CH 4 and O–O of O 2 are performed on a Rh 1 atom and thus CH 3 - and HO are formed on the Rh 1 atom. Insertion of C′O′ to Rh 1 –O bond of –Rh 1 –OH to form a –Rh 1 –C′O′OH on Rh 1 atom; the formed –Rh 1 –C′O′OH couples with CH 3 adsorbed on the same Rh 1 atom, generating the first product molecule, CH 3 C′O′OH. The left –Rh 1 =O activates the second CH 4 to form CH 3 and HO;   the formed CH 3 couples with CO to form acetyl, which couples with adsorbed HO to form the second acetic acid molecule. Preparation of isolated Rh catalytic site in ZSM-5 Rh cations were introduced to the internal surface of micropores of ZSM-5 through a method integrating vacuum pumping and incipient wetness impregnation (IWI). To minimize the amount of Rh cations to be deposited on external surface of a ZSM-5 particle, solution of Rh 3+ with the same volume as the pore volume of ZSM-5 was slowly dropped to ZSM-5 powder with a syringe pump when the catalyst powder was continuously stirred and remained in vacuum. During IWI, Rh cations exchanged with singly dispersed Brønsted acid sites of H-ZSM-5, which was prepared through calcining NH 4 -ZSM-5 at 400 °C for 12 h. After the introduction of Rh 3+ , the samples were further dried in an oven at 80 °C for 3 h and calcined in air at 550 °C for 3 h, forming the catalyst, Rh/ZSM-5. The evolution of the chemical environment of Rh cations in ZSM-5 was shown in Supplementary Fig. 1 . The concentration of Rh cations in the as-synthesized catalyst was measured through inductively coupled plasma atomic emission spectroscopy (ICP-AES). Before an ICP-AES measurement, 28 mg of 0.10 wt%Rh/ZSM-5 was dissolved in aqua regia. For catalyst with a nominal mass ratio of Rh to aliminosilicate, 0.10 wt%, the measured weight percent was 0.10 wt%, which suggests no obvious loss of Rh atoms during the preparation. X-ray photoelectron spectroscopy (XPS) studies of the as-synthesized 0.10 wt%Rh/ZSM-5 show the lack of Rh atoms in surface region of catalyst particles (red spectrum in Fig. 1c ). The lack of Rh atoms in surface region revealed with XPS together with the 0.10 wt%Rh in the as-synthesized catalyst measured with ICP-AES suggests that these introduced Rh atoms were anchored in micropores of ZSM-5 particles instead of the external surface of ZSM-5 particles. At a high loading (0.50 wt%Rh/ZSM-5), unfortunately rhodium oxide nanoparticles (2–4 nm) were formed as evidenced by the low contrast patches in transmission electron microscopy (TEM) image (Fig. 1b ), consistent with the observed Rh 3d photoemission feature in studies of sample using XPS (black spectrum in Fig. 1c ) [18] . Fig. 1 Structural characterization of isolated rhodium atoms in ZSM-5. a TEM image of particles of 0.10 wt%Rh/ZSM-5; scale bar: 10 nm. b TEM image of particles of 0.50 wt%Rh/ZSM-5; scale bar: 10 nm. c Rh 3d XPS peak of 0.l0 wt%Rh/ZSM-5 and 0.50 wt%Rh/ZSM-5. d Energy space of Rh K-edge of 0.l0 wt%Rh/ZSM-5 and Rh foil (reference sample) of X-ray absorption near edge spectra (XANES). e r-space of Rh K-edge of experimental (black) and calculated (red) data of the k 2 -weighted Rh K-edge EXAFS spectra of used 0.10 wt%Rh/ZSM-5. f Coordination number and bond length on average of the used 0.10 wt%Rh/ZSM-5. g r-space of Rh K-edge of experimental (black) and calculated (red) data of the k 2 -weighted Rh K-edge EXAFS spectra of Rh metal foil. h r-space of Rh K-edge of experimental (black) and calculated (red) data of the k 2 -weighted Rh K-edge EXAFS spectra of Rh 2 O 3 nanoparticles supported on Al 2 O 3 Full size image The existence of Rh atoms in the microproes of ZSM-5 after catalysis was confirmed by the measured concentration of Rh atoms remained in micropores with ICP-AES, which was 0.098 %. Extended X-ray absorption fine structure spectroscopy (EXAFS) was used to characterize the chemical environment of anchored Rh atoms of used 0.10 wt%Rh/ZSM-5 (the catalyst after reaction). After catalysis, the used catalyst powder was centrifuged and thus washed with deionized H 2 O several times and then dried in oven at 200 °C. The obtained powder was used for EXAFS studies in flowing He at 150 °C. r-space spectrum of K-edge of Rh atoms of the used catalyst show that Rh atoms bond with oxygen atoms and the average coordination number of oxygen atoms to a Rh atom is CN(Rh-O) of 5.23 ± 0.52 (Fig. 1e, f ). Notably, no contribution of Rh–Rh metal bonds was needed to fit the r-space spectrum of Rh K-edge (Fig. 1e ), suggesting that there is no evidence for formation of Rh–Rh metal bonds. This is consistent with the oxidization state of Rh shown in Fig. 1h . Similar to literature [19] , [20] , [21] , the second shell of rhodium oxide at 2.60 Å in r-space spectrum (Fig. 1h ) was clearly observed in our reference sample Rh 2 O 3 nanoparticles. However, there is lack of Rh–O–Rh peak at 2.60 Å in the r-space spectrum of 0.10 wt%Rh/ZSM-5 (black line in Fig. 1e ). It shows Rh atoms of our used catalyst do not have the second coordination shell of Rh atoms in terms of lack of Rh–O–Rh and thus there are no rhodium oxide nanoclusters formed in our used catalyst (0.10 wt%Rh/ZSM-5). Inspired by work of Gates group [14] , [22] , particularly the assignment of intensity at about 2.7 Å in r-space spectrum of Rh K-edge to Rh–O–Al with a Rh–(O)–Al distance of 3.02 Å [14] , [23] , [24] , [25] , we fit the small peak (α) at about 2.7 Å in Fig. 1e to Rh–O–Al. In addition, we fit the intensity at about 3.3 Å (β) in r-space of Rh K-edge to Rh–O–Si (Fig. 1e ); the coordination numbers of Al to Rh through O atom and Si to Rh through O atom are 1.55 ± 0.66 and 1.68 ± 0.71, respectively; the distances of Al and Si atoms to the Rh atoms are 3.168 ± 0.032 Å and 3.514 ± 0.072 Å, respectively. Thus, these EXAFS studies show that Rh atoms of 0.10 wt%Rh/ZSM-5 are singly dispersed in micropores of ZSM-5 and each Rh atom bond with about five oxygen atoms on average. In the following paragraphs, sometimes we used Rh 1 O 5 @ZSM-5 when we need to point out the coordination environment of the Rh atoms on average. Supplementary Fig. 1f schematically shows the structure of a catalytic site of Rh 1 O 5 anchored in micropores of ZSM-5. The replacement of Brønsted acid sites (BAS) of H-ZSM-5 by Rh cations was confirmed with 1 H NMR (nuclear magnetic resonance) of 0.10 wt%Rh/ZSM-5 and H-ZSM-5. As shown in Supplementary Fig. 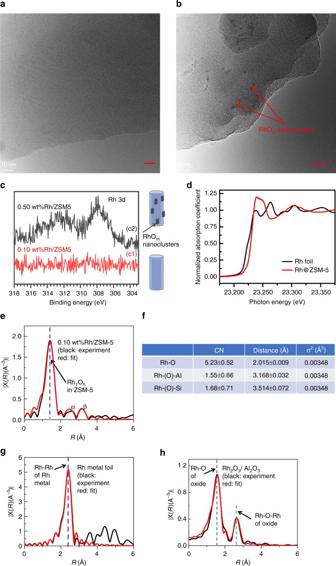Fig. 1 Structural characterization of isolated rhodium atoms in ZSM-5.aTEM image of particles of 0.10 wt%Rh/ZSM-5; scale bar: 10 nm.bTEM image of particles of 0.50 wt%Rh/ZSM-5; scale bar: 10 nm.cRh 3d XPS peak of 0.l0 wt%Rh/ZSM-5 and 0.50 wt%Rh/ZSM-5.dEnergy space of Rh K-edge of 0.l0 wt%Rh/ZSM-5 and Rh foil (reference sample) of X-ray absorption near edge spectra (XANES).er-space of Rh K-edge of experimental (black) and calculated (red) data of the k2-weighted Rh K-edge EXAFS spectra of used 0.10 wt%Rh/ZSM-5.fCoordination number and bond length on average of the used 0.10 wt%Rh/ZSM-5.gr-space of Rh K-edge of experimental (black) and calculated (red) data of the k2-weighted Rh K-edge EXAFS spectra of Rh metal foil.hr-space of Rh K-edge of experimental (black) and calculated (red) data of the k2-weighted Rh K-edge EXAFS spectra of Rh2O3nanoparticles supported on Al2O3 2a , the peak at 4.6 ppm was assigned to BAS site of H-ZSM-5 (Supplementary Table 1 ) [26] , [27] . It was not obviously observed in the same region of chemical shift in Supplementary Fig. 2b . This difference in Supplementary Fig. 2 suggests that the loss of some BAS sites due to ion exchange of Rh 3+ with H + in the IWI process. Catalytic performance of Rh 1 O 5 @ZSM-5 at 150 °C Catalytic activities of pure H-ZSM-5 and as-prepared Rh/ZSM-5 catalysts were measured by adding 28 mg catalyst to 10 mL deionized water in a Parr high-pressure reactor (Supplementary Fig. 3b ). The aqueous solution with dispersed catalyst particles was continuously, vigorously stirred by a magnetic bar coated with plastic materials at a speed of 600 rpm during catalysis. A mixture of CH 4 , CO, and O 2 with different partial pressure was introduced to the Parr reactor at room temperature. A portion of these reactant gases with a relatively high-pressure can diffuse to micropores of catalyst dispersed in the solvent (H 2 O or dodecane) and thus be catalyzed. Then, the reactor was heated to a set temperature. The reaction temperature of the solvent was directly measured through a thermocouple probe submerged to the solution consisting of the dispersed catalyst particles and solvent in the Parr reactor. The preservation of catalysis temperature for certain amount of time were performed by a temperature controller. This chemical transformation was performed for certain amount of time. The pressure, reaction temperature, and reaction time of each measurement of catalytic performance were given in the following figures and tables. Catalytic reaction under each condition was repeated at least four times. After each catalytic reaction, the solution in the Parr reactor consisting the used catalyst powder and liquid products was filtrated to separate the used catalyst powder. The clear liquid obtained after filtering the catalyst powder mainly contains acetic acid, methanol, formic acid, and solvent. The product solution was analyzed by 1 H NMR and 13 C NMR. The measurement was calibrated with 3-(trimethylsilyl)-1-propanesulfonic acid sodium salt (DSS) with chemical shift at δ = 0.0 ppm [11] , [28] . A DSS solution was prepared by dissolving DSS to D 2 O, making a solution with concentration of DSS in D 2 O at 0.020 wt%. Typically, 0.70 mL of the obtained clear liquid solution was mixed with 0.10 mL of as-prepared DSS solution in an NMR tube before NMR analysis. The identified oxygenate products were acetic acid ( δ = 2.08 ppm), formic acid ( δ = 8.28 ppm) and methanol ( δ = 3.33 ppm). A solvent suppression program was applied for minimizing the signal originating from H 2 O, similar to our previous studies [11] , [28] . Supplementary Fig. 4 is a representative NMR spectrum of solution after catalysis; peak of DSS was marked on it. To quantify the amounts of products, standard curves of acetic acid, formic acid, and methanol were carefully established and shown in Supplementary Fig. 5 . The analysis was described in the Methods section. 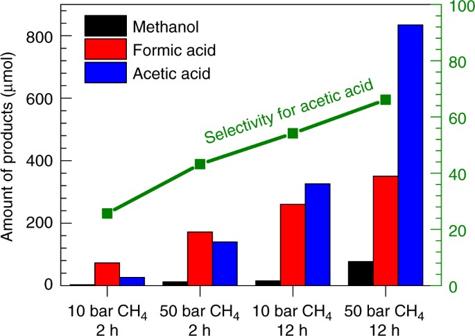Fig. 2 Catalytic performance of 0.10 wt%Rh/ZSM-5. Yields of acetic acid, formic acid and methanol as well as the selectivity to acetic acid as a function of different pressures of CH4(10 or 50 bars) and different reaction times (2 h or 12 h). 28 mg  of 0.10 wt%Rh/ZSM-5 was used for each catalysis test. Each catalysis test used 10 bar CO and 8 bar O2and certain pressure of CH4as noted onx-axis (10 or 50 bars). The catalysis temperatures of all studies here were 150 °C With 28 mg of 0.10 wt%Rh/ZSM-5, 226.1   μmol of total products (acetic acid, formic acid, and methanol) were produced at 150 °C in the first hour (entry 4 in Supplementary Table 2 ). Under the same condition, unfortunately the yields of the total organic compounds formed from 0.50 wt%Rh/ZSM-5 (entry 5 in Supplementary Table 2 ) are similar to 0.10 wt%Rh/ZSM-5. The similarity in catalytic performances of the two catalysts shows that the rhodium oxide nanoparticles formed on the surface of 0.50 wt%Rh/ZSM-5 are not active for this transformation. In other words, the catalytic activity of 0.10 wt%Rh/ZSM-5 in the production of acetic acid was contributed from the Rh 1 O 5 sites anchored in micropores of ZSM-5 instead of rhodium oxide nanoparticles supported on the external surface of ZSM-5. As the conversions of CH 4 in these studies of Fig. 2 and Table 1 are lower than 20%, we used these conversions and yields to calculate the turn-over rates with the equation: 
    TOR = Number of produced moelcules/Time of catalytic reaction ( S ) ×Number of acitve sites  ( Rh_1O_5 )
 (1) Fig. 2 Catalytic performance of 0.10 wt%Rh/ZSM-5. Yields of acetic acid, formic acid and methanol as well as the selectivity to acetic acid as a function of different pressures of CH 4 (10 or 50 bars) and different reaction times (2 h or 12 h). 28 mg  of 0.10 wt%Rh/ZSM-5 was used for each catalysis test. Each catalysis test used 10 bar CO and 8 bar O 2 and certain pressure of CH 4 as noted on x -axis (10 or 50 bars). The catalysis temperatures of all studies here were 150 °C Full size image Table 1 Comparison of TOR for formation of acetic acid or oxygenates including acetic acid, formic acid and methanol on 0.10 wt%Rh/ZSM-5 Full size table This calculation is based on an assumption that all loaded Rh atoms are active sites. This calculation was further described in Supplementary Methods. The activities for production of acetic acid and total organic oxygenates including acetic acid, methanol and formic acid at 150 °C are 0.070 and 0.10 molecules per Rh atom per second (entry 2 of Table 1 ), respectively. To check whether Rh atoms anchored in micropores of ZSM-5 could detach from ZSM-5, the clear solution was obtained by filtration for removal of Rh/ZSM-5 catalyst particles from the solution after catalysis at 150 °C for 12 h. ICP-AES test of this solution shows that only 2% of the total Rh atoms of 28 mg of 0.10 wt%Rh/ZSM-5 detached from ZSM-5 to solution. Thus, most Rh atoms remained in ZSM-5 after catalysis. Due to the negligible amount of Rh 3+ detached from 0.10 wt%Rh/ZSM-5 and the extremely low TOF of free Rh 3+ in solution evidenced in entry 3 in Table 1 , contribution of the detached Rh 3+ to the measured catalytic activity in formation of acetic acid is negligible. It suggests that the anchored Rh atoms are the active sites. To further confirm the contribution of Rh 1 O 5 sites to the formation of acetic acid, control experiments were performed on these catalysts including 28 mg of H-ZSM-5, 28 mg of 0.10 wt%Rh/SiO 2 and 28 mg of 0.10 wt%Rh/Al 2 O 3 under the exactly same condition as that of 28 mg 0.10 wt%Rh/ZSM-5 at 150 °C in the mixture of 10 bar CH 4 , 10 bar CO and 8 bar O 2 for 4 h. As shown in Table 2 , the amounts of acetic acid, formic acid, or methanol produced on 28 mg of 0.10 wt%Rh/SiO 2 and 28 mg of 0.10 wt%Rh/Al 2 O 3 are lower than 10 μmol, which are at the level of error bar. All the reported yields in this communication are the measured products formed from 28 mg catalyst. The yield could be shown as μmol/gram catalyst by multiplying a factor of \(\frac{{1000\;{\rm mg}/{\rm gram}}}{{28\;{\rm mg}}}\) . For example, the measured yields of methanol and acetic acid on 28 mg of 0.10%Rh/SiO 2 are 8.70 and 6.13 μmol, respectively; if they are multiplied by the factor \(\frac{{1000\;{\rm mg}/{\rm gram}}}{{28\;{\rm mg}}}\) they seem to indicate that 310 μmol methanol and 218 μmol acetic acid could form from one gram of 0.10%Rh/SiO 2 catalyst. Here, the multiplication is not meaningful since the values in Table 2 are at the uncertainty level. As the measured 8.70 μmol methanol and 6.13 μmol acetic acid from 28 mg 0.10%Rh/SiO 2 catalyst are in the range of error bar of these measurements, these values are not used to predict activity of 1 gram to compare with other catalysts. Even if the multiplication factor were applied, the activity of 0.10%Rh/SiO 2 is significantly lower than 0.10 wt%Rh/ZSM-5. For instance, 218 μmol acetic acid from per gram 0.10%Rh/SiO 2 calculated from the measured 6.13 μmol acetic acid per 28 mg is still much lower than 5000 μmol acetic acid from per gram 0.10 wt%Rh/ZSM-5 calculated from the measured 140 μmol acetic acid per 28 mg catalyst. In conclusion, these control samples in terms of Rh supported on these nonporous oxides and even on a couple of commonly used reducible oxides are not active for the production of acetic acid or methanol from coupling of CH 4 with CO and O 2 . Thus, these studies suggest the significant contribution of Rh 1 O 5 sites encapsulated in ZSM-5 to the formation of acetic acid. Table 2 Catalytic performances of 28 mg catalysts of 0.10 wt%Rh supported on different supports in a mixture of 10 bar CH 4 , 10 bar CO, and 8 bar O 2 at 150 °C for 3 h with 10 mL H 2 O in a high-pressure reactor Full size table The participation of all these three reactants (CH 4 , CO, and O 2 ) was confirmed with three parallel studies on 0.10 wt%Rh/ZSM-5 under the exactly same catalytic condition as listed in Supplementary Fig. 6a , b, c; in each of these studies, only two of the three reactants were introduced to the Parr reactor; none of these studies produced acetic acid, formic acid, or methanol due to the lack of the third reactant gas. Those studies clearly show that all the three gases (CH 4 , CO, and O 2 ) are necessary reactants for the formation of CH 3 COOH. The necessity of the three reactants was supported by DFT calculations described later. Participation of molecular O 2 in synthesis of acetic acid Here, we used low-cost molecular oxygen (O 2 ) or compressed air as oxidant in oxidative transformation of CH 4 and CO to acetic acid. To further confirm the direct participation of molecular O 2 , we performed catalysis at different pressures of O 2 (2, 4, 8, 12, and 16 bar) but all other conditions are the same in these parallel studies; in each of these parallel studies, 28 mg of 0.10 wt%Rh/ZSM-5 was added to 10 mL H 2 O. The reaction was performed at 150 °C for 2 h in a mixture of 35 bar CH 4 , 10 bar CO and different pressures of O 2 , in order to investigate the correlation of yields of products (acetic acid, formic acid, and methanol) with pressure of O 2 . As shown in Fig. 3a , highest yields of acetic acid and formic acid were obtained from the catalysis using 8 bar O 2 . The increase of yield of acetic acid and formic acid along the increase of O 2 pressure shows that O 2 does participate in the formation of acetic acid and formic acid. It is expected that high coverage of oxygen atoms on a Rh atom achieved with high-pressure O 2 could saturate Rh 1 atom with oxygen atoms, which poisons catalytic sites and thus results in a low yield of oxygenates at high pressure of O 2 . Fig. 3 Influence of partial pressure O 2 , CO and CH 4 on catalytic performances. Yields of methanol (black), formic acid (blue), and acetic acid (red) in the chemical transformation of CH 4 at 150 °C in aqueous solutions at different pressure of O 2 , CO, CH 4 . a 35 bar CH 4 , 10 bar CO, and different pressure of O 2 at 150 °C for 2 h. b 50 bar CH 4 , 8 bar O 2 , and different pressure of CO at 150 °C for 1.5 h. c 10 bar CO, 8 bar O 2 and different pressure of CH 4 at 150 °C for 2 h Full size image Direct participation of CO to synthesis of acetic acid To further confirm the participation of CO in the formation of acetic acid, influence of the partial pressure of CO on both the conversion of CH 4 and selectivity for production of acetic acid was investigated through parallel studies (Fig. 3b ). In each of these studies, the partial pressures of CH 4 and O 2 were fixed at 50 and 8 bar, respectively. However, the pressures of CO in the five studies are 2, 5, 10, 15, and 30 bar. The increase of the amount of acetic acid while CO pressure was increased from 2 to 10 bar suggests that CO directly participates into the formation of acetic acid. However, the lack of activity for production of acetic acid at 30 bar CO showed that catalyst sites were blocked at such a high-pressure of CO. Clearly, CO molecules must have directly interacted with the Rh cations. At high-pressure of CO, high coverage of CO could saturate the coordination of a Rh 1 atom and thus deactivate this catalyst. We measured the concentrations of Rh in the liquid (α) after filtration of the catalyst experienced the catalysis at 10 bar CO, 50 bar CH 4 , and 8 bar O 2 for 2.5 h, and in another liquid (β) after filtration of the catalyst experienced the catalysis at 30 bar CO, 50 bar CH 4, and 8 bar O 2 . The amounts of Rh atoms in the liquids α and β are 2.0% and 13.0% of all Rh atoms of 28 mg of 0.10 wt%Rh/ZSM-5, respectively. Thus, the much larger loss of Rh atoms at high-pressure of CO (30 bar) suggests that Rh atoms formed carbonyl in CO at high-pressure and some of these formed rhodium carbonyl species desorbed from micropores and then dissolved in the solution. Thus, some Rh species detached at high pressure of CO. A molecular-level evidence on direct participation of CO in the synthesis of acetic acid is the following isotope experiment. 0.7 bar 13 CO (Aldrich, 99%, total pressure 2.5 bar) was mixed with 6.3 bar of CO, 14 bar CH 4, and 8 bar O 2 for catalysis of 10 h (Fig. 4a ). As the chemical shift of 13 CH 3 OH in 13 C spectrum can be readily distinguished from acetic acid and formic acid, 40 μmol of 13 CH 3 OH (Aldrich, 99 at%) was added to the collected solution after catalysis as a reference to quantify the amount of potential isotope products 13 CH 3 COOH, CH 3 13 COOH, or H 13 COOH. As the unlabeled CO gas has a natural abundance of 13 C of 1.10%, a small amount of CH 3 13 COOH or H 13 COOH can form from the natural 1.10% 13 CO of unlabeled CO gas tank. Contrast experiments using the mixture of 7 bar of CO, 14 bar CH 4 , and 8 bar O 2 were performed (Fig. 4b ). The intensity ratio of the formed CH 3 13 COOH to 13 CH 3 OH in the solution of isotope experiment using 13 CO (Fig. 4a ) is obviously larger than those formed in the contrast experiment using unlabeled CO (Fig. 4b ) by 6.4 times; in addition, the intensity ratio of H 13 COOH to 13 CH 3 OH in isotope experiment (Fig. 4a ) is higher than that in the contrast experiment by 2.6 times (Fig. 4b ). They suggested that the C′ atoms of CH 3 C′OOH and HC′OOH came from C′O molecules. Notably, the intensity ratio of 13 CH 3 COOH to reference ( 13 CH 3 OH) in isotope experiment (Fig. 4a ) is the same as the ratio of the contrast experiment (Fig. 4b ). It suggests that the C atoms of CH 3 of CH 3 COOH do not come from the reactant CO. Fig. 4 13 C NMR studies of reaction using 13 CO or 13 CH 4 . 13 C NMR spectra of products of acetic acid, formic acid, and methanol on 28 mg 0.10 wt%Rh/ZSM-5 at 170 °C for 10 h in gas of a mixture of 0.7 bar 13 CO, 6.3 bar CO, 14 bar CH 4, and 8 bar O 2 , b mixture of 7 bar CO, 14 bar CH 4 , and 8 bar O 2 , c mixture of 7 bar CO, 0.7 bar 13 CH 4 , 13.3 bar CH 4 , and 8 bar O 2 , and d mixture of 7 bar CO, 14 bar CH 4 , and 8 bar O 2 . a and b are isotope experiments; c and d are their corresponding contrast experiments Full size image One potential pathway to form acetic acid is the coupling of CO with a formed formic acid molecule; if so, yield of acetic acid should increase along the increase of CO pressure. However, as shown in Fig. 3b yield of acetic acid decreases along with the increase of CO pressure (≥10 bar). Thus, coupling formic acid with CO to form acetic acid is not a pathway. To further check the possibility of reaction between HCOOH and CO to form acetic acid, we performed three control experiments at 150 °C for 3 h under the following conditions including mixture of 28 mg 0.10 wt%Rh/ZSM-5, 108 μmol HCOOH, and 10 mL DI H 2 O without any CO, mixture of 28 mg 0.10 wt%Rh/ZSM-5, 108 μmol HCOOH, and 10 mL DI H 2 O with 5 bar CO, and mixture of 28 mg 0.10 wt%Rh/ZSM-5, 108 μmol HCOOH, and 10 mL DI H 2 O with 10 bar CO. As shown in Supplementary Fig. 7 , no acetic acid was formed in these experiments. Direct participation of CH 4 in formation of CH 3 COOH The influence of CH 4 pressure on the catalytic performance was explored at 150 °C under a mixture of 10 bar CO and 8 bar O 2 and different pressure of CH 4 (10, 20, 30, 40, and 50 bar) for 2 h (Fig. 3c ). The progressive increase of yield of acetic acid along the increase of CH 4 pressure shows that CH 4 directly participates into the formation of acetic acid (Fig. 3c ), which excluded a pathway in which CH 4 couples with formic acid to form acetic acid. If acetic acid were formed from a coupling of formic acid with CH 4 , the amount of formic acid should have decreased along the increase of pressure of CH 4 since more formic acid should have been consumed along with the increased amount of CH 4 . To elucidate the source of carbon atoms at the molecular level, 13 CH 4 isotope experiments were performed. 0.7 bar 13 CH 4 (Aldrich, 99 at%) was mixed with 13.3 bar of CH 4 , 7.0 bar CO, and 8.0 bar O 2 for isotope experiment on 28 mg of 0.10 wt%Rh/ZSM-5 at 170 °C for 10 h (Fig. 4c ). A control experiment using 14 bar unlabeled CH 4 was performed under the exactly same catalytic condition (Fig. 4d ). 13 CH 3 COOH were formed in the two experiments. However, their ratio of 13 CH 3 COOH to reference ( 13 CH 3 OH) when 13 CH 4 was used (Fig. 4c ), is much larger than that when unlabeled CH 4 was used (Fig. 4d ). This difference shows that the carbon atom of CH 3 of acetic acid comes from CH 4 instead of CO. If C atoms of C=O of CH 3 COOH could come from CH 4 , the ratio of CH 3 13 COOH to reference ( 13 CH 3 OH) in Fig. 4c would be much larger than the ratio in Fig. 4d since the experiment of Fig. 4d contains significant amount of 13 CH 4 . In fact, in both experiments (Fig. 4c, d ), we did observe small amount of CH 3 13 COOH but there is no difference between their ratios to reference ( 13 CH 3 OH) in the experiments of both Fig. 4c, d . Here, the formation of CH 3 13 COOH is due to the natural abundance of 13 CO in unlabeled CO. Thus, CO does not contribute to the formation of CH 3 of CH 3 COOH. Direct coupling of reactants for formation of acetic acid It is noted that the amounts of the observed methanol in any of our studies of this work are always much lower than acetic acid and formic acid. One potential argument for the low yield of methanol could be that methanol has been formed but it could have acted as an intermediate compound in the formation of acetic acid; in other words, formic acid  could have been consumed through coupling with CO to form acetic acid. Depending on whether CH 3 OH could act as an intermediate product in the formation of acetic acid or not, two categories of potential pathways α and β were proposed in  Fig. 5a . In potential pathway α, CH 4 couples with CO to directly form acetic acid; methanol is not an intermediate product of this type of reaction pathway. In potential pathway β, however, CH 3 OH is an intermediate product and then be consumed in the formation of acetic acid; CH 4 is first oxidized to CH 3 OH (the first step) and then CH 3 OH couples with CO to form acetic acid (the second step); the second step of the potential pathway β is called carbonylation of methanol by CO; it is in fact the Monsanto process [29] , [30] , [31] . In order to identify whether CH 3 OH carbonylation (pathway β) could be a pathway for the production of acetic acid on our catalyst Rh 1 O 5 @ZSM-5, carefully designed isotope experiments described in Supplementary Methods were performed. Fig. 5 Isotope studies for elucidating whether acetic acid could be formed through coupling methanol with CO. a Two potential pathways α and β for production of acetic acid; in pathway α, CH 3 OH is not an intermediate compound for formation of CH 3 COOH; in pathway β, CH 3 OH is an intermediate compound  for formation of CH 3 COOH. b Potential catalytic products formed from 0.10 wt%Rh/ZSM-5 in the mixture of 13 CH 3 OH and H 2 O in solution under mixture of CH 4 , CO, and O 2 if the transformation of CH 4 , CO, and O 2 follows pathway α, β, or both α and β. c NMR spectra of the products formed from 28 mg of 0.10 wt%Rh/ZSM-5 after reaction in 10 bar CH 4 , 5 bar CO, and 4 bar O 2 at 150 °C for 1 h; there was no any isotope-labeled methanol, 13 CH 3 OH added to the rector before this catalysis test. d NMR spectra of the products formed from 28 mg of 0.10 wt%Rh/ZSM-5 after reaction in 10 bar CH 4 , 5 bar CO, and 4 bar O 2 at 150 °C for 1 h.; notably, 1.0 mmol 13 CH 3 OH was added to H 2 O before this catalysis test Full size image These isotope experiments show that acetic acid cannot be formed from carbonylation of methanol by CO on our catalyst. In one isotope-labeled experiment, 1.0 mmol isotope-labeled 13 CH 3 OH (99 atom% 13 C, Aldrich) was added to 10 mL deionized H 2 O before introduction of 10 bar CH 4 , 5 bar CO, and 4 bar O 2 to the Parr reactor. If CH 3 OH could not be an intermediate for formation of acetic acid, the added 13 CH 3 OH would not particulate into the formation of isotope-labeled acetic acid, 13 CH 3 COOH. Thus, no 13 CH 3 COOH could be observed if carbonylation of methanol by CO would not be involved (possibility 1 in Fig. 5b ). The NMR spectrum of the solution of products formed in the reactor having 12 CH 4 , 12 CO, and O 2 in H 2 O ( 13 CH 3 OH was not added) after reaction of 2 h was presented in Fig. 5c . Figure 5d is the NMR spectrum of the products formed after the catalysis for 1 h under a condition of mixture of 13 CH 3 OH, 12 CH 4 , 12 CO, and O 2 at 150 °C. The observed peaks A, B, C, D, and E in Fig. 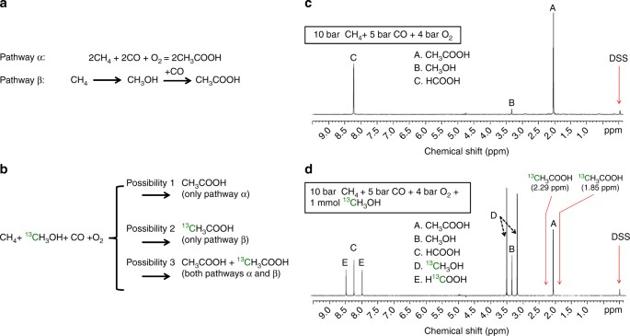Fig. 5 Isotope studies for elucidating whether acetic acid could be formed through coupling methanol with CO.aTwo potential pathways α and β for production of acetic acid; in pathway α, CH3OH is not an intermediate compound for formation of CH3COOH; in pathway β, CH3OH is an intermediate compound  for formation of CH3COOH.bPotential catalytic products formed from 0.10 wt%Rh/ZSM-5 in the mixture of13CH3OH and H2O in solution under mixture of CH4, CO, and O2if the transformation of CH4, CO, and O2follows pathway α, β, or both α and β.cNMR spectra of the products formed from 28 mg of 0.10 wt%Rh/ZSM-5 after reaction in 10 bar CH4, 5 bar CO, and 4 bar O2at 150 °C for 1 h; there was no any isotope-labeled methanol,13CH3OH added to the rector before this catalysis test.dNMR spectra of the products formed from 28 mg of 0.10 wt%Rh/ZSM-5 after reaction in 10 bar CH4, 5 bar CO, and 4 bar O2at 150 °C for 1 h.; notably, 1.0 mmol13CH3OH was added to H2O before this catalysis test 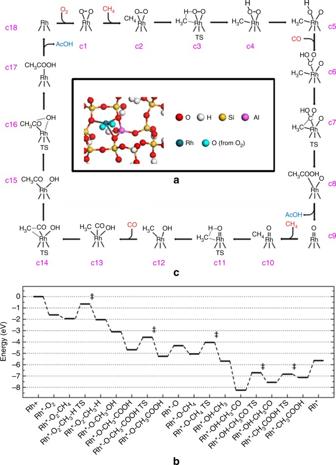Fig. 6 Computational studies of reaction pathway. Minimum-energy paths and reaction schematic for formation of acetic acid from CH4, CO, and O2on Rh1O5/ZSM-5. The formation of acetic acid is illustrated in a catalytic cycle starting with the singly dispersed Rh1O5site. The balanced reaction cycle consumes one O2, two CH4, and two CO to make two CH3COOH molecules (2CH4+2CO+O2=2CH3COOH).aThe optimized catalytic sites, Rh1O5anchored on Brønsted site in microspore of ZSM-5.bEnergy profile for pathway of transforming CH4, CO, and O2to CH3COOH.cIntermediates and transition states for a complete catalytic cycle, starting with Rh1O5(c1). Transition states are highlighted with the double dagger symbols 5d were assigned to CH 3 COOH, CH 3 OH, HCOOH, 13 CH 3 OH, and H 13 COOH, respectively. As neither peak of H atoms of 13 CH 3 of 13 CH 3 COOH in 1 H spectrum nor peak of 13 C atoms of CH 3 13 COOH in 13 C spectrum was observed in the NMR, pathway β is not a pathway for formation of acetic acid. Thus, these isotope studies showed that acetic acid is not formed from carbonylation of methanol by CO. Additionally, H 13 COOH was observed clearly in Fig. 5d , suggesting that 13 CH 3 OH can be oxidized to H 13 COOH under the current catalytic condition. We also performed the dry reforming of CH 4 by CO 2 by introducing 30 bar CH 4 and 30 bar CO 2 to the reactor containing 10 mL H 2 O and well dispersed 28 mg of 0.10 wt%Rh/ZSM-5. The reactor was heated to 150 °C and remained at 150 °C for 5 h and then cooled to 10 °C in ice water. As shown in Supplementary Fig. 6d , NMR test shows none of these products (acetic acid, formic acid, and methanol) was formed. Ready separation of products from hydrophobic solvent The above chemical transformation was performed in aqueous solution. As the products of this chemical transformation, acetic acid, formic acid, and methanol are hydrophilic, it is not readily to separate these hydrophilic products from water. To make these hydrophilic products automatically separate from solvent after synthesis, a hydrophobic solvent, n -dodecane was used. As shown in Supplementary Fig. 8 28 mg 0.10 wt%Rh/ZSM-5 in 10 mL n -dodecane in the mixture of 30 bar CH 4 , 10 bar CO, and 5 bar O 2 is definitely active for the formation of acetic acid. The significant advantage of using the hydrophobic solvent is that the hydrophilic products of this reaction including acetic acid, methanol, and formic acid can be readily separated from the hydrophobic solvent, without or with a low energy cost. Feature of this mild oxidation of methane in solution CH 4 and CO can be oxidized with different oxidants including O 2 , concentrated H 2 SO 4 , or a superacid [32] , [33] , [34] by using homogeneous catalyst [32] , in which acetic acid and other products (formic acid and methanol) were formed. One control experiment using Rh(NO 3 ) 3 was done (entry 3 in Table 1 ); the turn-over-rate (TOR) of the homogenous catalyst, Rh(NO 3 ) 3 without a promoter is only 6.3 × 10 −6 molecules per rhodium cation per second at 150 °C. Here, the Rh 1 O 5 @ZSM-5 catalyzes the oxidation of CH 4 and CO with a low-cost oxidant, molecular oxygen or even air at 150 °C at a solid–liquid–gas interface. TOR of the catalytic sites Rh 1 O 5 anchored in microporous silicate reaches 0.070 CH 3 COOH molecules on per Rh 1 O 5 site per second in mixture of 50 bar CH 4 , 10 bar CO, and 8 bar O 2 (entry 2 of Table 1 ). These TORs for production of acetic acid on singly dispersed site Rh 1 O 5 are much higher than those reported homogenous catalysts [32] , [33] by >1000 times. As shown in Fig. 2 , 840 μmol of acetic acid, 352 μmol of formic acid, and 82 μmol of methanol were produced from 28 mg 0.10 wt%Rh/ZSM-5 at 150 °C for 12 h under a catalytic condition of 50 bar CH 4 , 10 bar CO and 8 bar O 2 , which correspond to conversion of 10.2% of CH 4 under this condition. Selectivity for production of acetic acid among all organic products reaches about 70% under this condition. Other than the highest catalytic efficiency on Rh 1 O 5 @ZSM-5, a significant advantage of our catalytic process is the ready separation of liquid products from the solid catalyst and solvent. It is found that a shorter reaction time gives a higher selectivity for formation of formic acid and a longer reaction time lead to a higher selectivity for formation of acetic acid. As shown in Supplementary Fig. 9 both formic acid and acetic acid are the main products when reaction time is shorter than 3 h. When the reaction time is 3 h or longer, acetic acid is the main product. The evolution of the yields of formic acid and acetic acid as a function of time implies that the relative low temperature of catalyst in the heating from 25 to 150 °C is favorable for the formation of formic acid. More discussion on time-dependent selectivity for formation of formic acid and acetic acid can be found from Supplementary Discussion. Understanding reaction mechanism at molecular level Based on the coordination environment of Rh 1 atoms suggested by EXAFS studies, we used a structural model whose Rh atom bonds with three oxygen atoms of the substrate wall and two oxygen atoms of one oxygen molecule in our computational studies. Our DFT calculations suggest that the Rh atom prefers a ten-membered-ring channel, which has smaller repulsion, instead of a six-membered ring channel of ZSM-5. Based on the experimental preparation method, we expect that the Rh 1 cations replace the Bronsted sites and thus bind to the Al atoms. As shown in Fig. 6a this Rh 1 atom binds to three oxygen atoms of the Si–O framework and two oxygen atoms of reactant, making Rh 1 exhibit positive to 0.927 |e|. Fig. 6 Computational studies of reaction pathway. Minimum-energy paths and reaction schematic for formation of acetic acid from CH 4 , CO, and O 2 on Rh 1 O 5 /ZSM-5. The formation of acetic acid is illustrated in a catalytic cycle starting with the singly dispersed Rh 1 O 5 site. The balanced reaction cycle consumes one O 2 , two CH 4 , and two CO to make two CH 3 COOH molecules (2CH 4 +2CO+O 2 =2CH 3 COOH). a The optimized catalytic sites, Rh 1 O 5 anchored on Brønsted site in microspore of ZSM-5. b Energy profile for pathway of transforming CH 4 , CO, and O 2 to CH 3 COOH. c Intermediates and transition states for a complete catalytic cycle, starting with Rh 1 O 5 (c1). Transition states are highlighted with the double dagger symbols Full size image Isotope experiments suggest two necessary steps: activation of C–H bond of CH 4 to form CH 3 and insertion of CO to form acetic acid. Based on these experimental findings, reaction pathway on the Rh 1 O 5 with lowest energy was simulated and transition states were located (Fig. 6 ). 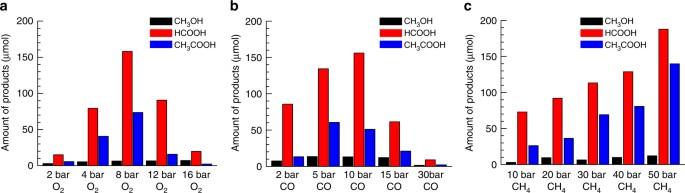The energy profile and catalytic cycle are illustrated in Fig. 6b, c , respectively. Fig. 3 Influence of partial pressure O2, CO and CH4on catalytic performances. Yields of methanol (black), formic acid (blue), and acetic acid (red) in the chemical transformation of CH4at 150 °C in aqueous solutions at different pressure of O2, CO, CH4.a35 bar CH4, 10 bar CO, and different pressure of O2at 150 °C for 2 h.b50 bar CH4, 8 bar O2, and different pressure of CO at 150 °C for 1.5 h.c10 bar CO, 8 bar O2and different pressure of CH4at 150 °C for 2 h The specific energies are listed in Supplementary Table 3 . We found that the Rh 1 O 5 active site (Fig. 6a ) participates in the reaction by first activating C–H bond of methane (c2 and c3) with an activation barrier of 1.29 eV. It forms a methyl and hydroxyl adsorbed on the Rh atom (c4). Then, a CO molecule can insert to the Rh–O bond of Rh–O–H, forming a COOH adsorbed on Rh (c6). Then COOH can couple with the adsorbed methyl with a barrier of 1.11 eV (c7), forming a weakly adsorbed acetic acid (c8). Subsequent desorption yields the first CH 3 COOH molecule. The remaining Rh-O oxo group (c9) activates C–H bond of the second CH 4 molecule to form a methyl and a hydroxyl group adsorbed on the Rh atom (c12). Following, or concurrently to this step, the second CO molecule binds to the unsaturated Rh site (c13). Then, the adsorbed CO inserts into the methyl–Rh bond with a barrier of 1.54 eV (c14), forming an acetyl group (c15). Finally, the hydroxyl group couples with carbon atom of C=O of the acetyl group to form the second acetic acid with a barrier of 0.72 eV (c17). Desorption of the second acetic acid molecule recovers the Rh site (c18), which then  bonds with a molecular O 2 , forming a Rh 1 O 5 site (c1) ready for next catalytic cycle. Our experimental studies show that high pressure of CO (Fig. 3b ) in fact decreased the activity for producing acetic acid and finally poisoned the active sites. Computational study explored the observed influence of CO pressure on the catalytic activity. It suggests that saturated coordination of Rh with CO molecules under CO gas at a high pressure can poison a Rh 1 site and thus prevent it from forming acetic acid. In addition, the DFT calculations show the activation energy for C – H of CH 4 is largely increased if the Rh 1 pre-adsorbed two CO molecules at high-pressure of CO (Supplementary Fig. 10b ). More information can be found in Supplementary Discussion. In summary, the heterogeneous catalyst, 0.10 wt%Rh/ZSM-5 consisting of singly dispersed Rh 1 O 5 sites anchored in the micropores of microporous aluminate silicate was prepared. The anchored Rh 1 O 5 sites exhibit unprecedented catalytic activity in synthesis of acetic acid higher than free Rh 3+ in aqueous solution by >1000 times under mild conditions. This heterogeneous catalytic process opens a new route to synthesize acetic acid through direct utilization of methane under a mild condition at 150 °C or lower  by using a low-cost oxidant, O 2 or air instead of current industrial process of synthesizing acetic acid through carbonylation of methanol. Preparation and characterization of catalyst Two steps were involved in the preparation of a Rh/ZSM-5 catalyst. The first step is the preparation of H-ZSM-5 by calcining zeolite NH 4 -ZSM-5 with a SiO 2 /Al 2 O 3 ratio of 23 (Alfa Aesar) in air at 400 °C for 12 h. Four Rh/ZSM-5 catalysts with different Rh concentrations (0.01 wt%, 0.05 wt%, 0.10 wt%, 0.50 wt%) were synthesized through a method integrating vacuum pumping and IWI of aqueous solution containing certain amount of rhodium(III) nitrate hydrate (~36% Rh basis, Sigma-Aldrich) at room temperature. Typically, 500 mg of H-ZSM-5 was placed in a 50 mL three-port flask. The three ports were sealed with three corks. One port was connected to a vacuum pump. Before injection of Rh(NO 3 ) 3 solution, air in the flask containing 100 mg H-ZSM-5 was purged for 3–5 h by a vacuum pump when the H-ZSM-5 powder was being stirred. The size of stirring bar is5 mm for maximizing the amount of H-ZSM-5 to be stirred. Then, 0.30 mL of 1.0 mg/mL Rh(NO 3 ) 3 aqueous solution was added to the H-ZSM-5, which had been pumped for 3–5 h. The injection needle quickly reached the powder to avoid the dispersion of solution to the wall of flask since the environment of flask is in vacuum. In addition, the tip of needle was buried in the middle of H-ZSM-5 powder during injection, minimizing diffusion of solution to the wall of flask. During the injection, the H-ZSM-5 should be continuously stirred. After the introduction of Rh 3+ , the samples were further dried in an oven at 80 °C for 3 h and calcined in air at 550 °C for 3 h. Supplementary Fig. 1 schematically shows the evolution of the structure of the anchored Rh atoms in ZSM-5 of 0.10 wt%Rh/ZSM-5. Actual Rh contents were determined by inductively coupled plasma atomic emission spectrometry (ICP-AES). TEM (FEI, Titan 80–300) was used to characterize the morphology of the catalyst. EXAFS of Rh K-edge was taken at SPring-8. For EXASF studies, the used catalyst of 0.10 wt%Rh/ZSM-5 was measured when the catalyst was kept at 150 °C in the flow of pure He. The adsorption fine structure spectra of Rh K-edge were fitted using IFEFFIT package and FEFF6 theory. Reference samples including Rh metal foil and Rh 2 O 3 nanoparticles supported on Al 2 O 3 were studied with EXAFS. Their r-space spectra of these reference samples were fitted with the same software. XPS was performed using a PHI5000 VersaProbe Spectrometer with monochromated Al Kα as X-ray source. Catalytic reactions Transformation of methane to acetic acid on 0.10 wt%Rh/ZSM-5 was performed in a Parr high-pressure reactor (Series 4790, Parr) containing a Teflon liner vessel (Supplementary Fig. 3b ). 28 milligram 0.10 wt%Rh/ZSM-5 was added to 10 mL H 2 O in the reactor. After evacuating the air left in reactor by flowing CH 4 (99.9%, Matheson) and purging for five times, the system was pressurized with reactant gases in a sequence of CH 4 , CO (99.9%, Matheson) and O 2 (99.9%, Matheson) to their desired pressures. The high-pressure reactor was completely sealed and then heated to the desired reaction temperature (typically 150 °C) by placing it in an oil bath. The temperature controller of the heating plate (VWR International) was used to measure the temperature of solution in the Parr reactor through the thermocouple placed in solution of Parr reactor and to control the temperature through outputting tunable power to the heating plate. Once the desired catalysis temperature was reached, the solution was vigorously stirred at 1200 rpm and was maintained at the reaction temperature for certain amount of time. After completion of the reaction, the vessel was cooled in an ice bath to a temperature below 10 °C to minimize the loss of volatile products. The solution with liquid products was filtered from the catalyst powder. The clean liquid containing acetic acid, formic acid, and methanol was analyzed by 1 H-NMR or 13 C-NMR. The concentration of Rh in the filtered powder was examined with ICP-AES as described in Supplementary Methods. Supplementary Fig. 11 is the standard curve of ICP-AES studies of Rh concentrations. Measurements of products with NMR and GC 1 H NMR spectra were collected at room temperature on a Bruker AVANCE III HD 400 spectrometer at University of Notre Dame and University of Kansas. The measurements were calibrated by using 3-(trimethylsilyl)-1-propanesulfonic acid sodium salt (DSS) residual signal at δ = 0.0 ppm. Supplementary Fig. 4 is a typically NMR spectrum of products formed from CH 4 transformation. Obviously, the peak of DSS can be identified. Typically, 0.7 mL collected filtrate and 0.1 mL of D 2 O (with 0.02 wt% DSS) were mixed in an NMR tube for analysis. The identified oxygenated products were acetic acid ( δ = 2.08 ppm), formic acid ( δ = 8.24 ppm) and methanol ( δ = 3.34 ppm). A solvent suppression program was applied in order to minimize the signal originating from H 2 O, similar to our previous studies [11] . To quantify the products, standard curves were built using the same method as that of our previous report [11] . To establish a standard curve of a specific product such as acetic acid, a series of standard solutions with different concentrations of acetic acid were prepared. For instance, to establish a standard curve acetic acid, a series of standard solutions with different concentrations of acetic acid were prepared. NMR spectra of these standard solutions were collected with the exactly same parameters of NMR measurements. The ratio of the area of peak of acetic acid ( δ = 2.08 ppm) to area of DSS of the same solution were calculated. These ratios of solutions with different concentrations of acetic acid were plotted as a function of the concentrations of acetic acid. This graph is a standard curve of acetic acid (Supplementary Fig. 5a ), formic acid (Supplementary Fig. 5b ), and methanol (Supplementary Fig. 5c ). Concentration of a product (such as acetic acid) in a solution after catalysis in Parr reactor was determined by locating the ratio of the peak area of the product to the area of DSS on the y -axis of the standard curve (such as Supplementary Fig. 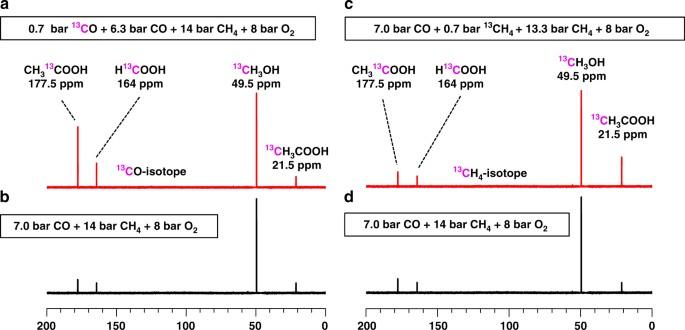5a ) and then finding the corresponding value on x -axis, which is the amount of the product of the solution after a catalysis in the unit of μmol. Gases in the head of Parr reactor after catalysis were analyzed with GC. Fig. 4 13C NMR studies of reaction using13CO or13CH4.13C NMR spectra of products of acetic acid, formic acid, and methanol on 28 mg 0.10 wt%Rh/ZSM-5 at 170 °C for 10 h in gas ofamixture of 0.7 bar13CO, 6.3 bar CO, 14 bar CH4,and 8 bar O2,bmixture of 7 bar CO, 14 bar CH4, and 8 bar O2,cmixture of 7 bar CO, 0.7 bar13CH4, 13.3 bar CH4, and 8 bar O2, anddmixture of 7 bar CO, 14 bar CH4, and 8 bar O2.aandbare isotope experiments;canddare their corresponding contrast experiments Supplementary Table 4 presents the amounts of all reactants before catalysis and all products and left reactants after the catalysis; this catalysis was performed on 28 mg 0.10 wt%Rh/ZSM-5 dispersed in 10 mL deionized H 2 O under 50 bar CH 4 , 10 bar CO, and 8 bar O 2 for  3 h. Bruker Topspin 3.5 software was used to acquire, process, and visualize the data. Data availability All data are available from the authors upon reasonable request